Chromoselective access toZ- orE- allylated amines and heterocycles by a photocatalytic allylation reaction The most useful strategies for the alkylation of allylic systems are related to the Tsuji–Trost reaction or the use of different Lewis acids. Herein we report a photocatalytic approach for the allylation reaction of a variety of nucleophiles, such as heteroarenes, amines and alcohols. This method is compatible with a large variety of pyrroles and indoles, containing different substituents such as electron-withdrawing and electron-donating groups, unprotected nitrogen atoms and bromo derivatives. Moreover, this methodology enables the chromoselective synthesis of Z - or E -allylated compounds. While the use of UV-light irradiation has allowed the synthesis of the previously inaccessible Z -allylated products, E -isomers are prepared simply by changing both the light source to the visible region, and the catalytic system. Based on mechanistic and photochemical proofs, laser flash photolysis studies and DFT calculations, a rational mechanism is presented. The preparation of allyl-substituted compounds has attracted a special interest due to their utility as building blocks in organic synthesis [1] , [2] , [3] . The Tsuji–Trost reaction [4] is one of the most powerful methodologies for the alkylation of allylic systems, which is commonly catalyzed by palladium, and the allylic position is usually activated by a halide, an acetate, or a carbonate (eq. a, Fig. 1 ) and affords exclusively the E- isomer. The high selectivity and the general scope of this reaction makes it one of the most prominent Csp 3 –Csp 3 bond formation methodologies [5] . Indoles and pyrroles are versatile and useful heterocycles for the synthesis of a large variety of biologically active compounds and natural products [6] . Different authors have reported the allylation of indoles at the C-3 position via the Tsuji–Trost reaction in a racemic manner [7] , [8] , [9] , [10] , [11] , [12] . However, although this methodology is very important, to the best of our knowledge, no photocatalytic approaches for the allylation of heterocycles have been reported so far. Fig. 1 The photocatalytic allylation reaction. a Precedents in the Tsuji–Trost allylation and b this work Full size image Over the past decade, photocatalysis has emerged as a powerful tool for the construction of new bonds that are difficult to obtain using other established procedures [13] , [14] , [15] , [16] , [17] , [18] , [19] , [20] , [21] , [22] , [23] , [24] , [25] , [26] , [27] , [28] , [29] , [30] , [31] . A large number of photocatalytic methodologies have been described for the formation of new Csp 2 –Csp 2 bonds. In particular, the arylation of (hetero)-aromatic rings, usually pyrroles, under different photocatalytic systems has been recently reported [32] , [33] , [34] , [35] , [36] , [37] , [38] , [39] , [40] . However, one of the major problems related to this photocatalytic arylation is the large excess of the heterocycle required in this reaction (24–40 equiv.). Although the photocatalytic heteroatomatic ring arylation has been extensively studied, the photoallylation of heterocycles remains an elusive process. We hypothesize that the reduction of the allylic derivative by a photocatalyst with the adequate redox potential would result in the appropriate intermediate, which will allow the functionalization of the allylic position. There are two prerequisites to achieve this goal: (i) the development of a photocatalytic system able to activate the C–O bond; (ii) since an unsaturation is present, it is necessary to control the isomerization of the double bond ( Z or E ). In this work, we present a chromoselective photocatalytic allylation of heteroaromatic rings, using smooth conditions and short reaction times to access the Z - or E -double bonds, depending on the reaction conditions (eq. b, Fig. 1 ). In addition, mechanistic and photochemical proofs, DFT calculations, and laser flash photolysis studies enabled us to postulate a plausible mechanistic pathway. Optimization of the model reaction Based on the previous photocatalytic arylation reactions [32] , [33] , [34] , [35] , [36] , [37] , [38] , [39] , [40] , we started the screening of the reaction using the acetate allylic derivative 1a and pyrrole 2a (18 equiv.) 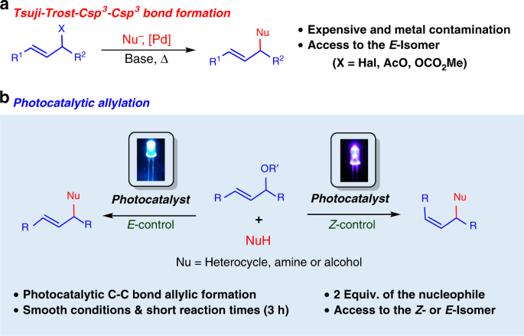Fig. 1 The photocatalytic allylation reaction.aPrecedents in the Tsuji–Trost allylation andbthis work in the presence of different photocatalysts 3 under light irradiation (Table 1 ). Transition-metal-based photocatalysts ( 3a–3b ) failed to promote the formation of the allylated heterocycle (entries 1 and 2). Several photoorganocatalysts with different reductive power ( 3c–3f ) were tested, but only the 10-phenyl-10 H -phenothiazine (PTH) ( 3e ) gave the Z- allylated pyrrole 4a with low conversion under 420-nm LED irradiation (entries 3–6). Encouraged by these results, we used an irradiation source with a wavelength closer to the maximum absorption of PTH (entry 7). Pleasantly, using a 365-nm LED, 4a was obtained with a 65% conversion. In the absence of a photocatalyst, light, and both, the allylation did not proceed (entries 8–10), confirming the photocatalytic nature of this transformation. Different solvents were then evaluated, and the best result was obtained using CH 3 CN (entries 7 and 11–14). In order to decrease the amount of heterocycle, the reaction was carried out using 10 and 2 equivalents of 2a (entries 15 and 16) and 4a was obtained with a good yield of 58% in only 3 h, using just two equivalents of the heterocycle. The use of inorganic bases (Na 2 CO 3 , LiOAc) afforded the final product, although with moderate yield, due to the lower solubility of such bases in acetonitrile (entries 17 and 18). 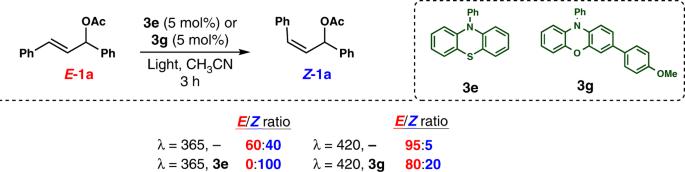Fig. 2 Isomerization studies. Isomerization proofs ofE-1aunder different catalysts (3eand3g) and different irradiation wavelengths Table 1 Optimization of the photocatalytic allylation reaction a Full size table Substrate scope Having established the best conditions (Table 1 , entry 16), we performed the scope of the reaction (Table 2 ). With N -methyl pyrrole, the allylic derivative 4b was obtained with a better yield than 4a and with a similar selectivity for the Z -isomer. Other substituents were tolerated at the N -atom of the pyrrole ( 4c and 4d ) with excellent Z / E selectivity (up to 96:4) and with a slight decrease for the phenyl derivative 4c . Indoles without protecting groups at the nitrogen were also employed, keeping the high selectivity for the Z -isomers, and with better yields than with the pyrroles (compare 4e and 4f with 4a and 4b ). Electron-donating groups (EDGs) were well tolerated at different positions of the indole ring ( 4g , 4h, and 4i ) as well as electron-withdrawing groups (EWG) at the aromatic ring ( 4j ). A methyl substituent next to the indolinic nitrogen ( 4k ) or the reactive C-3 center ( 4l ) did not have a negative influence on the reactivity, obtaining both in very good yields and high selectivity. Remarkably, the presence of Br at the 5-position ( 4m ) was also well tolerated under the presence of the high-reducing photocatalyst 3e . The scope of the allylic derivative was also evaluated. Electron-rich ( 4n , 4o, and 4p ) as well as electron-poor aromatic rings ( 4q ) worked with excellent selectivities (up to > 98:2). We then studied the influence of the leaving group at the allylic position (R group in 1a ). The reaction worked with other leaving groups such as benzoate, carbamate, or carbonate, which were suitable for this process. However, the reaction with the hydroxyl group did not proceed, because of its higher reduction potential (−2.52 V vs. SCE) compared with the other activated allylic alcohols (E = −2.06 to −2.35 V vs. SCE, see Suplementary Note 4 for cyclic voltammetry). Table 2 Scope of the allylation reaction for the synthesis of Z -isomers with pyrroles and indoles under catalyst 3e a,b Full size table After obtaining these good results with the Z -isomer, our next objective was the development of a photocatalytic variant to obtain the corresponding E -isomers. To achieve this goal, we analyzed the conditions that avoided the isomerization of the reagent 1a . A sample containing E - 1a in MeCN was irradiated for 3 h under different reaction conditions (Fig. 2 ). Without the use of the photocatalyst under 365-nm irradiation, we found a mixture of 60/40 E / Z - 1a , while in the presence of 3e , this isomerization to Z - 1a was complete (Fig. 2 ). According to theoretical calculations, photosensitization and subsequent isomerization of E - 1a by the photocatalyst is feasible, while photosensitization and subsequent isomerization of Z - 1a cannot take place (see Supplementary Information Fig. 25 ). The absorption spectra of E - 1a at the reaction conditions revealed a significant absorption at 365 nm (see Supplementary Information Fig. 8 ), while at 420 nm, it was negligible, suggesting that the reaction must be carried out in the visible-light region to avoid isomerization. Under 420-nm irradiation, only 5% of the E - 1a was isomerized to the Z -isomer after 3 h. Therefore, a photocatalyst with high reduction potential (≥2.35 V vs. SCE) and absorption in the visible-light region is required. The phenoxazine 3g , that meets all these criteria [41] , resulted in only a small amount of Z - 1a at 420-nm irradiation after 3 h (Fig. 2 ). Therefore, under these conditions (using photocatalyst 3g and 420-nm irradiation), it should be possible to avoid the isomerization step and selectively form E -allylated products 5 . Fig. 2 Isomerization studies. 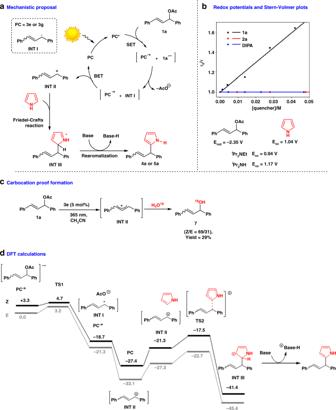Fig. 3 Mechanistic studies.aMechanistic proposal for the photoallylation.bRedox potentials and Stern–Volmer plots of the time-resolved fluorescence quenching of3gwith1a, pyrrole, and DIPA (DIPA = diisopropylamine).cReaction of1awith H2O18under standard reaction conditions.dFor DFT calculations, geometry optimizations were performed using the M06-2X functional in combination with the 6-311G** basis set Isomerization proofs of E - 1a under different catalysts ( 3e and 3g ) and different irradiation wavelengths Full size image To our delight, when carrying out the reaction between the allylic derivative 1a and pyrrole ( 2a ) in the presence of the photocatalyst 3g under 420-nm irradiation, the allylated product E - 5a was obtained with a good yield as the major isomer (Table 3 ). Other N -substituted pyrroles were also employed and maintained the same selectivity ( 5b–5c ). Only compound 5d was obtained as a complex mixture. The reaction with indoles afforded even better yield and selectivity than pyrroles ( 5e and 5f ). Unprotected indolinic nitrogen as well as different substituents were tolerated, from EDGs ( 5g–i ) to EWGs ( 5j ), methyl ( 5k–l ), or bromo derivatives ( 5m ), obtaining in all cases good yields (67–92%) and excellent selectivities (up to > 98:2). The isomerization of the final product 5e under 420-nm irradiation was also studied, obtaining a Z/E mixture 30/70 after 3 h of irradiation, without the photocatalyst, while in the presence of the photocatalyst 3g, a Z/E mixture 20/80 was obtained. The final product is present in the reaction in higher concentrations only after 2 h of reaction. Therefore, the irradiation time is not enough to produce its isomerization, which explains the obtention of the E -isomer as the major one. Table 3 Scope of the allylation reaction for the synthesis of E -isomers with pyrroles and indoles under catalyst 3g a,b Full size table Mechanistic studies The proposed reaction mechanism is outlined in Fig. 3a . After light absorption by the photocatalyst under LED irradiation ( λ = 365 or 420 nm), single-electron transfer (SET) takes place from its S 1 excited state ( E S1 = 3.2 eV, see Supplementary Information Figs. 11 and 12 ) to 1a . Steady-state and time-resolved fluorescence quenching studies in the presence of 1a afforded a quenching rate constant of k q (S 1 ) = 4.7 × 10 9 M −1 s −1 (see Supplementary Information Fig. 9a ), indicating that the radical ion pair ( PC •+ + 1a •− ) formation occurs at nearly diffusion rate. In addition, SET from the excited singlet state would be an exergonic process, taking into account the free energy change (Δ G ET = −4.0 kcal mol −1 ) associated with the electron transfer (see Supplementary Note 4 for Rehm–Weller equation). Fig. 3 Mechanistic studies. a Mechanistic proposal for the photoallylation. b Redox potentials and Stern–Volmer plots of the time-resolved fluorescence quenching of 3g with 1a , pyrrole, and DIPA (DIPA = diisopropylamine). c Reaction of 1a with H 2 O 18 under standard reaction conditions. d For DFT calculations, geometry optimizations were performed using the M06-2X functional in combination with the 6-311G** basis set Full size image Importantly, photooxidation of DIPEA ( E ox = 0.94 V vs. SCE) [42] , DIPA ( E ox = 1.17 V vs. SCE) [43] , or pyrrole ( E ox = 1.04 V vs. SCE) [44] by PC S 1 excited state could not occur, taking into account the oxidation power of 3e and 3g ( E (Pc*/Pc·−) = −0.3 V vs. SCE for 3e and 3g , see Supplementary Note 4 ), and was further confirmed by fluorescent-quenching studies (see Fig. 3b ). The fate of such reduced species has been investigated by DFT calculations, considering both Z- and E -isomers (Fig. 3d ). Initial single-electron transfer process from the photocatalyst ( PC ) to 1a generates the radical cation PC ·+ and the radical anion 1a · − , that evolves through the C–O bond scission to afford acetate anion and the radical intermediate I ( INT I ). This step is a very exergonic process (−22 or −21.3 kcal mol −1 ) and proceeds through a very shallow kinetic barrier ( E a = 1.4 or 3.2 kcal mol −1 ). Then, the oxidation of INT I by the oxidized photocatalyst ( PC ·+ ), results in the regeneration of the photocatalyst ( PC ) and formation of a carbocationic intermediate II ( INT II ) (Fig. 3d ). Such electron transfer is calculated as a thermodynamically favorable process (−8.7 or −11.8 kcal mol −1 ). The calculated energetic barriers for E to Z isomerizations for radical or carbocation intermediates I and II rule out this process from such transient species (see Supplementary Information Fig. 28 ). Formation of this carbocation INT II was experimentally confirmed, carrying out the reaction in the presence of H 2 O 18 as the nucleophile obtaining the isotopically labeled compound 7 (Fig. 3c ). In addition, when two nonsymmetric allylic derivatives bearing different aryl groups were studied, an equimolecular mixture of products was obtained (see Supplementary Fig. 30 , compounds 6 and 6′ ), indicating that the reaction takes places through a common intermediate. Then, a Friedel–Crafts reaction between the carbocation INT II and pyrrole takes place, generating the protonated intermediate III ( INT III ). This step is also theoretically found exergonic (−14 or −26.3 kcal mol −1 ) and kinetically favorable ( E a = 3.8 kcal mol −1 ). A final rearomatization by deprotonation of INT III gives the final product (Fig. 3d ). For such deprotonation, both DIPEA and the anion acetate (formed during the reaction) would act as a base through very exergonic processes (see entries 16 and 17 from Table 1 for reactions in the presence of Na 2 CO 3 and LiOAc). In order to gain a better understanding of the reaction mechanism, laser flash photolysis (LFP) measurements have been carried out. Excitation of 3g at 355 nm results in two peaks at 468 and 530 nm at 40 ns after the laser pulse, which are assigned to the 3g radical cation ( 3 g •+ ) and the excited triplet state of 3g ( 3 3g* ), respectively (Fig. 4a , black line, for further details, see also Supplementary Note 2 ). This experiment was performed in the presence of 1a to identify the possible transient reaction intermediates (Fig. 4a , red line). Two new absorption bands at 360 and 490 nm are clearly observed, which correspond to intermediates I and II , respectively, based on literature data [45] . The lifetime of the carbocation INT II also depends on the nucleophilicity of the anionic leaving group (see Supplementary Information Fig. 4 ). In order to check whether formation of INT II and INT I is instantaneous with the laser pulse, additional LFP experiments of 3g in the presence of increasing amounts of 1a were performed (Fig. 4c and d ). Generation of INT II is practically instantaneous even at lower concentration of 1a (Fig. 4d ), whereas lifetimes of INT I are not affected by higher amounts of 1a (Fig. 4c ). This result suggests that SET from 3g * to 1a at diffusion control rate (see Supplementary Information Fig. 9 ) gives rise to the contact radical ion pair at this singlet stage (Fig. 3a ). All processes in the contact radical ion pairs undergo in the sub-nanosecond scale [46] . Fast acetate release from 1a · − led to INT I , which is still in close contact with 3g •+ . At this point, INT I undergoes an ultrafast back electron transfer with 3g •+ restoring 3g and generating INT II, whose amount is slightly dependent on the concentration of 1a in the sample (Fig. 4d ). In addition, 3g •+ and INT I can split up, forming the corresponding free 3g •+ and free INT I , that are detected in the LFP experiments with lifetimes in the microsecond scale (Fig. 4a , red line). Once the detection of both intermediates I and II by LFP has been established, the question arises whether INT I or INT II (radical or carbocation) would react with a trapping agent (Fig. 4e and transient absorption spectrum in Fig. 4b ). Addition of pyrrole to a 3g / 1a mixture results only in a marked decrease of the INT II lifetime (Fig. 4g ), while the band corresponding to INT I (360 nm) is not affected (Fig. 4f ). Therefore, this experiment clearly corroborated with the previous data (Fig. 3 ) that the carbocation INT II is the reactive intermediate in our reaction. A quantum yield of 1.5% was found, suggesting a photocatalytic process without a significant radical chain propagation [47] . Fig. 4 Laser flash photolysis ( λ exc = 355 nm, MeCN/Ar) experiments. a Transient absorption spectra recorded at 40 ns after the laser pulse of 3g (50 mM) without 1a (black), with 70 mM of 1a (red). b Transient absorption spectra recorded at 40 ns after the laser pulse of 3g (50 mM) with 70 mM of 1a (black) and with 35 mM of 2a (red). c Decay kinetics at 360 nm after 355-nm LFP of 3g (50 µM) in the presence of increasing amounts of 1a . d Decay kinetics at 485 nm after 355-nm LFP of 3g (50 µM) in the presence of increasing amounts of 1a . e Scheme of the formation of intermediate II from intermediate I and their reaction with 2a . f Lifetime of INT I : decays monitored at 360 nm of 3g (50 mM) and 1a (70 mM) (black line) and in the presence of 2a (37 mM) (red line). g Lifetime of INT II : decays monitored at 490 nm of 3g (50 mM) and 1a (70 mM) (black line) and in the presence of 2a (37 mM) (red line) Full size image Scope with alcohols and amines Once that we proved that the reaction takes place through a carbocation intermediate formation, we decided to study other nucleophiles to prove the generality of our protocol. Allylic amines are very useful compounds that can be employed as building blocks for the synthesis of amino acids, alkaloids, and carbohydrate derivatives [48] , [49] , [50] . Moreover, this structure is present in numerous natural products and drugs with antifungal, antibacterial, and anti-inflammatory action [51] , [52] , [53] . 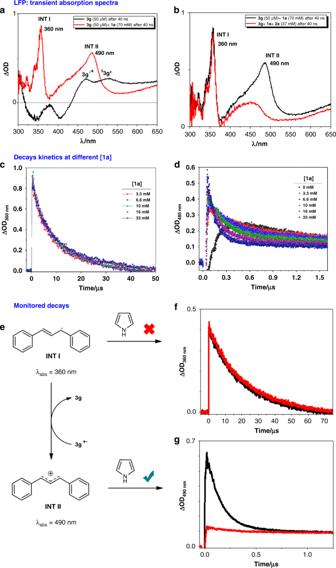Fig. 4 Laser flash photolysis (λexc= 355 nm, MeCN/Ar) experiments.aTransient absorption spectra recorded at 40 ns after the laser pulse of3g(50 mM) without1a(black), with 70 mM of1a(red).bTransient absorption spectra recorded at 40 ns after the laser pulse of3g(50 mM) with 70 mM of1a(black) and with 35 mM of2a(red).cDecay kinetics at 360 nm after 355-nm LFP of3g(50 µM) in the presence of increasing amounts of1a.dDecay kinetics at 485 nm after 355-nm LFP of3g(50 µM) in the presence of increasing amounts of1a.eScheme of the formation of intermediateIIfrom intermediateIand their reaction with2a.fLifetime ofINT I: decays monitored at 360 nm of3g(50 mM) and1a(70 mM) (black line) and in the presence of2a(37 mM) (red line).gLifetime ofINT II: decays monitored at 490 nm of3g(50 mM) and1a(70 mM) (black line) and in the presence of2a(37 mM) (red line) Different amines were tried under UV irradiation in order to obtain the Z -allylated amines which are not accessible by other methodologies (Table 4 ). Aniline gave the corresponding Z -allylated amine 9a with high selectivity. Aromatic amines with EDGs were well tolerated ( 9b–d ) with moderate selectivity, whereas anilines with EWGs gave significant better yield ( 9e ) and Z / E ratio. In addition, the presence of Br at the aromatic ring was tolerated without detecting the corresponding reduced product ( 9f ). Aliphatic primary and secondary amines were also suitable for the reaction conditions ( 9g–h ). Cyclic allylated amine 9i was obtained in good selectivity ( Z : E = 91:9) and good yield. Moreover, the use of morpholine as a nucleophile can be employed for the synthesis of 9j with excellent selectivity. The preparation of allylic ethers has a great interest, as they are also present in numerous pharmaceuticals and natural products [54] , [55] , [56] , [57] . For this reason, alcohols were employed as nucleophiles, obtaining Z -allylated ethers with good yields and good selectivities ( 9k–m ) [58] . Table 4 Scope of the allylation reaction with amines and alcohols for the synthesis of Z -isomers under photocatalyst 3e a,b Full size table Using the visible-light irradiation conditions and photocatalyst 3g with amines and alcohols is possible to obtain the corresponding E -isomers (Table 5 ). Aromatic amines gave the corresponding allylated compounds with high selectivities and good yields with EDGs ( 10b–d ) and EWGs ( 10e ), or ortho -bromo substituents ( 10f ). Aliphatic primary ( 10g ) and secondary amines ( 10h–j ) were employed, keeping in all the cases high Z / E selectivity. Moreover, allylated ethers can also be obtained under visible-light irradiation with excellent selectivities ( 10k–m ). A similar mechanistic scenario was found for amines and alcohols, using p -toluidine 8b as a nucleophile in the LFP and photochemical mechanistic probes (see Supplementary Fig. 9 ). Table 5 Scope of the allylation reaction with amines and alcohols for the synthesis of E -isomers under photocatalyst 3g a,b Full size table In summary, a chromoselective photocatalytic approach for the allylation of indoles, pyrroles, amines, and alcohols has been developed. This approach represents a photocatalytic allylation reaction for the synthesis of demand of Z - or E -isomers, with only two equivalents of the desired nucleophile. Therefore, under UV-light irradiation Z -allylated products are obtained, while the E -isomer is simply prepared by changing both the light source to the visible region, and the catalytic system. DFT calculations, photochemical proofs, and mechanistic experiments indicate that the most plausible mechanism involves a nucleophilic attack to an allyl-cation intermediate. Procedure for the preparation of Z -allylic compounds A vial equipped with a magnetic stir bar and fitted with a Teflon screw cap septum was charged with the corresponding allylic compound 1 (0.1 mmol), the corresponding heterocycle, amine, or alcohol (0.2 mmol), N -phenyl phenothiazine (1.4 mg, 5 mol%), DIPEA (86 μL, 0.5 mmol), and acetonitrile (1 mL). The reaction was degassed with three freeze–pump–thaw cycles. The vial was then backfilled with N 2 and stirred under 365-nm LED irradiation (8.2460 W m −2 intensity; approximate distance was 2 cm from the vial) at 20 °C. After 3 h, the vial was opened, the solvent evaporated, and the crude product was purified by column chromatography to give the corresponding products 4 or 9 . Procedure for the preparation of E -allylic compounds A vial equipped with a magnetic stir bar and fitted with a Teflon screw cap septum was charged with the corresponding allylic compound 1 (0.1 mmol), the corresponding heterocycle, amine, or alcohol (0.2 mmol), 3-(4-methoxyphenyl)-10-phenyl-10H-phenoxazine (1.7 mg, 5 mol%), DIPA (70 μL, 0.5 mmol, only base is needed for reactions with heterocycles as nucleophile), and acetonitrile (1 mL). The reaction was degassed with three freeze–pump–thaw cycles. The vial was then backfilled with N 2 and stirred under 420-nm LED irradiation (18.3396 W m −2 intensity; approximate distance was 2 cm from the vial) at room temperature. After 3 h, the vial was opened, the solvent evaporated, and the crude product was purified by column chromatography to give the corresponding products 5 or 10 .